Nanoscale nickel oxide/nickel heterostructures for active hydrogen evolution electrocatalysis Active, stable and cost-effective electrocatalysts are a key to water splitting for hydrogen production through electrolysis or photoelectrochemistry. Here we report nanoscale nickel oxide/nickel heterostructures formed on carbon nanotube sidewalls as highly effective electrocatalysts for hydrogen evolution reaction with activity similar to platinum. Partially reduced nickel interfaced with nickel oxide results from thermal decomposition of nickel hydroxide precursors bonded to carbon nanotube sidewalls. The metal ion–carbon nanotube interactions impede complete reduction and Ostwald ripening of nickel species into the less hydrogen evolution reaction active pure nickel phase. A water electrolyzer that achieves ~20 mA cm −2 at a voltage of 1.5 V, and which may be operated by a single-cell alkaline battery, is fabricated using cheap, non-precious metal-based electrocatalysts. Hydrogen, as a clean and renewable energy resource, has been intensely investigated as an alternative to the diminishing fossil fuel [1] , [2] , [3] , [4] . An effective way of producing high-purity hydrogen is to electrochemically split water into hydrogen and oxygen in an electrolyzer [5] , [6] , [7] , [8] , [9] , [10] . Nickel (Ni) and stainless steel are typically used in industry for water reduction and oxidation catalysis respectively in basic solutions [7] , [11] . However, Ni metal is not an ideal water reduction or hydrogen evolution reaction (HER) catalyst due to its high overpotential (~200 mV) and large Tafel slope [11] , [12] . The state-of-art HER catalyst is platinum (Pt) and its alloys, but the scarcity and cost of Pt limit its large-scale application for electrolysis [13] . Active and stable non-precious metal-based HER catalysts in alkaline solutions have been pursued [14] , [15] , [16] , [17] , [18] , [19] , [20] , [21] , [22] , [23] including Raney Ni [16] , [17] and Nickel molybdenum (NiMo) alloy [14] , [15] , [18] , [19] , [21] . It remains difficult to achieve both high activity and stability matching those of Pt. Here, we report a nickel oxide/nickel (NiO/Ni) hetero-junction-like structure attached to mildly oxidized carbon nanotube (NiO/Ni-CNT) exhibiting high HER catalytic activity close to commercial Pt/C catalysts in several types of basic solutions (pH=9.5–14). The NiO/Ni nano-hybrids is fabricated serendipitously in a low-pressure thermal annealing experiment, affording partial reduction of nickel hydroxide (Ni(OH) 2 ) coated on oxidized CNTs that acts as an interacting substrate to impede complete reduction and aggregation of Ni. The high catalytic activity of NiO/Ni-CNT towards HER enables a high-performance electrolyzer with ~20 mA cm −2 at a voltage of 1.5 V. Synthesis and characterization of NiO/Ni-CNT catalyst NiO/Ni-CNT synthesis was done by low-temperature hydrolysis of Ni salts into Ni hydroxide on the sidewalls of mildly oxidized CNT [Ni(OH) 2 /ox-CNT], followed by a low-pressure (~1.5 torr) annealing at 300 °C in an Ar flow. The synthesis was very simple and could be easily scaled up for practical use. Scanning transmission electron microscopy (STEM) images revealed the presence of ~10 nm nanoparticles attached to multi-walled CNT ( Fig. 1a,b ). Chemical mapping with electron energy-loss spectroscopy (EELS) resolved the distribution of O, Ni and C with sub-nm spatial resolution, identifying a core shell-like structure with O and Ni in the shell and only Ni in the core ( Fig. 1d–f ) over a CNT network. High-resolution STEM imaging ( Fig. 1b and Supplementary Fig. 1 ) and the corresponding chemical mapping ( Fig. 1d ) showed that the NiO shell was not uniform, containing small NiO grains with different orientations and might contain small gaps in the shell to expose some NiO/Ni nano-interfaces ( Fig. 1c ). 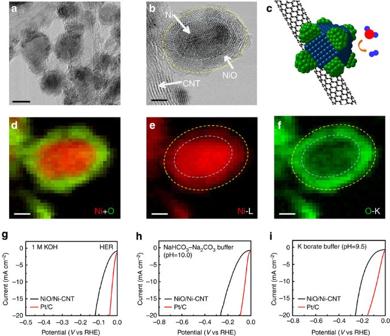Figure 1: Structure and performance of a highly active NiO/Ni-CNT nano-hybrid. (a) Low-magnification STEM bright-field image showing the typical morphology of the NiO/Ni-CNT sample, with 8–15 nm particles attached to CNTs. Scale bar, 2 nm. (b) Atomic resolution STEM bright-field image showing the structure of a typical NiO/Ni particle on a CNT (small NiO nanoparticles over a larger Ni nanoparticle core). Scale bar, 2 nm. (c) A schematic illustration of the NiO/Ni-CNT structure. Scale bar, 2 nm. (d–f) Chemical maps for the spatial distribution of Ni and O and their overlay, from the whole area shown inb. The two dashed circles highlight the NiO particle layer on the surface of the Ni core. Scale bar, 2 nm. (g–i) Linear sweep voltametry of NiO/Ni-CNT and Pt/C ing1 M KOH (h) NaHCO3-Na2CO3buffer (pH=10.0) and (i) potasium borate buffer (pH=9.5) at a scan rate of 1 mV s−1under the loading of 0.28 mg cm−2on RDE showing high HER catalytic activity of NiO/Ni-CNT. Figure 1: Structure and performance of a highly active NiO/Ni-CNT nano-hybrid. ( a ) Low-magnification STEM bright-field image showing the typical morphology of the NiO/Ni-CNT sample, with 8–15 nm particles attached to CNTs. Scale bar, 2 nm. ( b ) Atomic resolution STEM bright-field image showing the structure of a typical NiO/Ni particle on a CNT (small NiO nanoparticles over a larger Ni nanoparticle core). Scale bar, 2 nm. ( c ) A schematic illustration of the NiO/Ni-CNT structure. Scale bar, 2 nm. ( d – f ) Chemical maps for the spatial distribution of Ni and O and their overlay, from the whole area shown in b . The two dashed circles highlight the NiO particle layer on the surface of the Ni core. Scale bar, 2 nm. ( g – i ) Linear sweep voltametry of NiO/Ni-CNT and Pt/C in g 1 M KOH ( h ) NaHCO 3 -Na 2 CO 3 buffer (pH=10.0) and ( i ) potasium borate buffer (pH=9.5) at a scan rate of 1 mV s −1 under the loading of 0.28 mg cm −2 on RDE showing high HER catalytic activity of NiO/Ni-CNT. Full size image X-ray photoelectron spectroscopy (XPS) confirmed the NiO-Ni structure ( Supplementary Fig. 2a ). The as-made material exhibited mostly Ni 2+ species on the surface with a weak shoulder peak at ~853 eV from Ni 0 . On Ar ion sputtering of the surface, the detected Ni species were mostly Ni 0 with decreased amount of Ni 2+ , consistent with NiO-decorated Ni nanoparticles. The Ni K edge spectrum of the sample recorded by X-ray absorption near edge spectroscopy (XANES) further corroborated the co-existence of NiO and Ni ( Supplementary Fig. 2b ). Since Ni K edge probed deeper into the material, we could estimate the Ni/NiO ratio ~73/27 by linear fitting of standard patterns. The HER catalytic property of NiO/Ni-CNT was measured in a three-electrode configuration by with a rotating disk electrode (RDE) at 1,600 r.p.m. to remove H 2 bubbles generated. Commercial Pt/C was investigated side-by-side under the same loading of 0.28 mg cm −2 . In 1 M potassium hydroxide (KOH), the NiO/Ni-CNT afforded little overpotential at low current density with only a slightly lower current increase compared to Pt/C and a Tafel slope of 82 mV per decade ( Fig. 1g and Supplementary Fig. 3a ). Impressively, the NiO/Ni-CNT catalyst achieved an HER current density of 10 mA cm −2 at <100 mV overpotential. Moreover, high-performance HER catalysis by NiO/Ni-CNT was also observed in a carbonate/bicarbonate buffer (pH=10.0) and a borate buffer (pH=9.5; Fig. 1h,i ). Synergistic effects of NiO and Ni on HER catalysis When annealed at 300 °C at a higher Ar pressure of 1 atm (in contrast to~1.5 torr for producing NiO/Ni-CNT), the same Ni(OH) 2 precursors on CNTs was transformed to pure 3–4 nm NiO nanoparticles (NiO/CNT; Fig. 2b and Supplementary Fig. 4 ), suggesting no Ni 2+ reduction under a high annealing pressure with the release of oxygen gas. On the other hand, Ni 2+ reduction was accelerated by raising the annealing temperature to 500 °C in ~1.5 torr Ar, generating Ni nanoparticles (mostly>10 nm particles) nearly free of NiO on CNTs (Ni/CNT; Fig. 2c and Supplementary Fig. 4 ). The Ni surface oxidation state on NiO/CNT and Ni/CNT were confirmed to be +2 and 0, respectively, by XPS and XANES spectra ( Fig. 2g,h ) and by EELS chemical mapping ( Fig. 2e,f and Supplementary Figs 5 and 6 ). 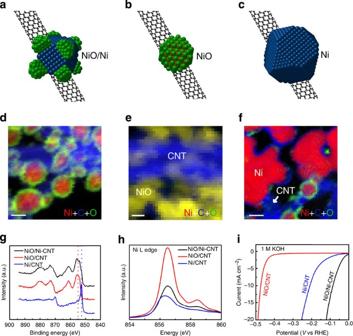Figure 2: Structure and performance of NiO/Ni-CNT compared with NiO/CNT and Ni/CNT. (a–c) Schematic illustrations of (a) NiO/Ni-CNT, (b) NiO/CNT and (c) Ni/CNT structure. (d–f) Reconstructed elemental maps with Ni in red, C in blue and O in green for (d) NiO/Ni-CNT, scale bar is 5 nm (e) NiO/CNT, scale bar is 2 nm and (f) Ni/CNT structure, scale bar is 10 nm. (g) High-resolution Ni XPS spectra of the three hybrid materials (the dotted line points out the binding energy of Ni2+(red) and metallic Ni (blue). (h) Ni L edge XANES spectra of the three hybrid materials. (i) Linear sweep voltametry of the three hybrid materials in 1 M KOH at a scan rate of 1 mV s−1under the loading of 0.28 mg cm−2on RDE showing superior HER catalytic activity of NiO/Ni-CNT. Figure 2: Structure and performance of NiO/Ni-CNT compared with NiO/CNT and Ni/CNT. ( a – c ) Schematic illustrations of ( a ) NiO/Ni-CNT, ( b ) NiO/CNT and ( c ) Ni/CNT structure. ( d – f ) Reconstructed elemental maps with Ni in red, C in blue and O in green for ( d ) NiO/Ni-CNT, scale bar is 5 nm ( e ) NiO/CNT, scale bar is 2 nm and ( f ) Ni/CNT structure, scale bar is 10 nm. ( g ) High-resolution Ni XPS spectra of the three hybrid materials (the dotted line points out the binding energy of Ni 2+ (red) and metallic Ni (blue). ( h ) Ni L edge XANES spectra of the three hybrid materials. ( i ) Linear sweep voltametry of the three hybrid materials in 1 M KOH at a scan rate of 1 mV s −1 under the loading of 0.28 mg cm −2 on RDE showing superior HER catalytic activity of NiO/Ni-CNT. Full size image The NiO/CNT material afforded a much larger overpotential of ~400 mV, despite a smaller Tafel slope and CNT alone showed negligible HER current density before −0.5 V versus RHE ( Supplementary Fig. 7 ). The Ni/CNT hybrid gave similar Tafel slope in HER but a larger overpotential of ~130 mV than the ~0 mV overpotential for NiO/Ni-CNT. This advantage was partially attributed to the higher surface area of NiO/Ni-CNT (152.2 m 2 g −1 ) compared with that of Ni/CNT (86.5 m 2 g −1 ; Supplementary Fig. 8a ). With current density normalized to the surface area instead of the geometric area, NiO/Ni-CNT still outperformed Ni/CNT by ~100 mV ( Supplementary Fig. 8b ). Further, we compared the HER activity of a physical mixture of Ni/CNT and NiO/CNT with Ni/CNT alone, without observing any difference and both were inferior to NiO/Ni-CNT ( Supplementary Fig. 9 ). These results suggested that the HER catalytic activity might be facilitated by a synergistic effect between NiO and Ni. Important role of CNT in NiO/Ni heterostructure synthesis It is interesting that the formation of NiO/Ni heterostructure relied on the oxidized CNT growth substrate. Without any CNT as support, the same reaction steps produced aggregated Ni particles in a plate-like morphology ( Fig. 3a ) with lower HER activity than NiO/Ni-CNT ( Fig. 3b and Supplementary Fig. 10 ), in strong contrast to the small nanoparticle structure of NiO/Ni on CNT ( Fig. 3a ). NiO/Ni heterostructures growing on oxidized CNT with different oxidation degree showed similar HER catalytic activity in 1 M KOH ( Supplementary Fig. 11 ). These results suggested that on oxidized CNTs, the reduction of oxidized Ni species during thermal decomposition was impeded or retarded likely due to pinning or interactions of Ni species with oxidized CNTs through oxygen functional groups, delaying the reduction of Ni into larger aggregates via Ostwald ripening. This result was observed serendipitously and underscored that substrate–precursor interaction could profoundly affect the morphology, structure and catalytic activity of materials. 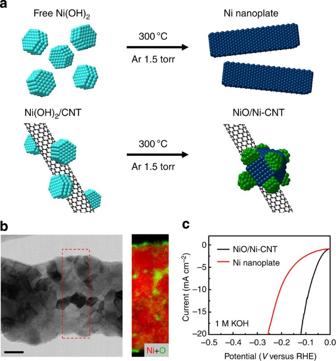Figure 3: Different products made by the same reaction with and without oxidized CNT. (a) A schematic illustration of the structural difference between CNT hybrid and pure nanoparticle (b) STEM BF image showing the typical morphology of the CNT-free Ni nanoplate and the corresponding reconstructed maps from the highlighted area with Ni in red and O in green. Only a very small amount of NiO particles is observed on the surface. Scale bar, 20 nm. (c) Linear sweep voltametry of NiO/Ni-CNT hybrid and CNT-free Ni nanoplate in 1 M KOH at a scan rate of 1 mV s−1under the loading of 0.28 mg cm−2on RDE. Figure 3: Different products made by the same reaction with and without oxidized CNT. ( a ) A schematic illustration of the structural difference between CNT hybrid and pure nanoparticle ( b ) STEM BF image showing the typical morphology of the CNT-free Ni nanoplate and the corresponding reconstructed maps from the highlighted area with Ni in red and O in green. Only a very small amount of NiO particles is observed on the surface. Scale bar, 20 nm. ( c ) Linear sweep voltametry of NiO/Ni-CNT hybrid and CNT-free Ni nanoplate in 1 M KOH at a scan rate of 1 mV s −1 under the loading of 0.28 mg cm −2 on RDE. Full size image Water electrolysis by NiO/Ni-CNT and NiFe LDH Towards electrolysis applications, we loaded the NiO/Ni-CNT material into Ni foam at a high loading of ~8 mg cm −2 (based on mass of NiO/Ni). The HER catalytic activity of the electrode was high in 1 M KOH, showing <100 mV overpotential at a current density of 100 mA cm −2 and an impressively low Tafel slope of 51 mV per decade ( Fig. 4a and Supplementary Fig. 3 , please refer to Supplementary Fig. 12 for uncompensated curve, Supplementary Fig. 13 for mean value and s.d. of applied potential at certain current densities and Supplementary Table 1 for comparison with other representative HER electrocatalysts). There was only a slight difference in the activity between NiO/Ni-CNT and precious metal Pt/C catalyst (~20 mV @ 20 mA cm −2 and ~50 mV @ 100 mA cm −2 ). Compared with bare Ni foam that resembled Ni foil used in industrial water splitting, the NiO/Ni-CNT electrode afforded a gain of ~200 mV lower in voltage ( Fig. 4a ). Similar gain of ~300 mV over Ni foam was obtained in bicarbonate–carbonate buffer and borate buffer electrolytes, respectively ( Supplementary Fig. 14a,b ). In addition, the constant current curves of NiO/Ni-CNT at HER region exhibited good stability to maintain a high HER current density of 20 mA cm −2 over the course of 2 h in all three electrolytes ( Supplementary Fig. 14c ). 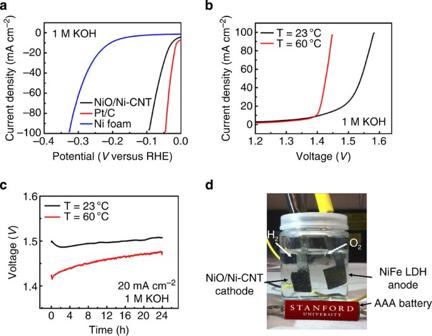Figure 4: High-performance NiO/Ni-CNT cathode for water splitting with a single battery. (a) Linear sweep voltametry of NiO/Ni-CNT, Pt/C deposited on Ni foam and pure Ni foam at a scan rate of 1 mV s−1under the loading of 8 mg cm−2in 1 M KOH. For uncompensated curve, please refer toSupplementary Fig. 10. (b) Linear sweepment voltametry of water electrolysis using NiO/Ni-CNT as HER catalyst and NiFe LDH as OER catalyst (both loaded into Ni foam at a loading of 8 mg cm−2based on the active mass) in 1 M KOH under different temperature. (c) Chonopotentiometry of water electrolysis using NiO/Ni-CNT and NiFe LDH at a constant current density of 20 mA cm−2in 1 M KOH. (d) Demonstration of water-splitting device powered by an AAA battery with a nominal voltage of 1.5 V. Figure 4: High-performance NiO/Ni-CNT cathode for water splitting with a single battery. ( a ) Linear sweep voltametry of NiO/Ni-CNT, Pt/C deposited on Ni foam and pure Ni foam at a scan rate of 1 mV s −1 under the loading of 8 mg cm −2 in 1 M KOH. For uncompensated curve, please refer to Supplementary Fig. 10 . ( b ) Linear sweepment voltametry of water electrolysis using NiO/Ni-CNT as HER catalyst and NiFe LDH as OER catalyst (both loaded into Ni foam at a loading of 8 mg cm −2 based on the active mass) in 1 M KOH under different temperature. ( c ) Chonopotentiometry of water electrolysis using NiO/Ni-CNT and NiFe LDH at a constant current density of 20 mA cm −2 in 1 M KOH. ( d ) Demonstration of water-splitting device powered by an AAA battery with a nominal voltage of 1.5 V. Full size image We made an electrolyzer using NiO/Ni-CNT as water reduction catalyst and a high-performance NiFe-layered double hydroxide (NiFe LDH) water oxidation catalyst [28] . The experiment was carried out in 1 M KOH at room temperature (~23 °C) and~60 °C. Water electrolysis with low current density of 20 mAcm-2 at ~1.50 V and high current density of 100 mAcm-2 at ~1.58 V was observed at room temperature ( Fig. 4b ). Notably, this was the first time ever reported to achieve a voltage of <1.5 V for water electrolysis using non-precious catalysts for both electrodes. Such water electrolysis could be powered by a single-cell AAA battery with a nominal voltage of ~1.5 V ( Fig. 4d and see Supplementary Movie 1 for a movie of water electrolysis by an AAA battery). The kinetics and thermodynamics were greatly improved at high temperature (~60 °C), showing lower voltage of ~1.42 V at 20 mA cm −2 and higher current increase, reaching 100 mA cm −2 at a voltage of ~1.45 V ( Fig. 4b ) with good stability ( Fig. 4c and Supplementary Fig. 15 ). The result suggested that the NiO/Ni heterostructure catalyst could match the benchmark Pt/C catalyst for efficient electrolyzers with ultralow overpotential for water-splitting devices. Due to the observation of gaps in the NiO shell and thus incomplete coverage of the Ni core by NiO, we proposed that the exposed NiO/Ni nano-interfaces might be synergistically active sites for HER catalysis. In alkaline media, the HER pathway could be through the Volmer–Heyrovsky process or Volmer–Tafel pathways [24] , [25] . Both pathways involve the adsorption of H 2 O molecule, electrochemical reduction of adsorbed H 2 O into adsorbed OH − and H atom, desorption of OH − to refresh the surface and formation of H adsorbed intermediate for H 2 generation. Ni metal has been calculated to have a suitable H atom binding energy close to Pt (refs 26 , 27 ), but is much worse in HER catalytic activity compared with Pt. Therefore, we tentatively propose that the formation and desorption of OH − might be an important step for HER in alkaline condition. On a NiO/Ni interface, the OH − generated by H 2 O splitting could preferentially attach to a NiO site at the interface due to strong electrostatic affinity to the locally positively charged Ni 2+ species and more unfilled d orbitals in Ni 2+ than Ni metal, while a nearby Ni site would facilitate H adsorption and thus the Volmer process, imparting synergistic HER catalytic activity to NiO/Ni. A pure NiO surface is not active for HER due to the lack of H adsorption sites. On a pure Ni surface without any NiO, the adsorbed OH − species could occupy the sites for H atom, causing inefficient release of OH − and blocking of the active catalytic sites. Admittedly, detailed mechanistic insights into electrocatalysis of the heterostructure NiO/Ni material are currently limited partly due to difficulties in theoretical modelling by density functional theory of HER processes in basic solutions involving charged species participating in the reactions. Future work will address this challenge and perform in situ spectroscopic techniques to glean the reaction mechanisms and pinpoint the HER active sites in the NiO/Ni material. In summary, we discovered nanoscale NiO/Ni heterostructure attached to CNT network as a novel HER catalyst. The structure of Ni cores partially covered with small NiO nanoparticles was created by a simple process of Ni(OH) 2 decomposition involving CNT substrate delaying the Ni(OH) 2 reduction and Ni aggregation. An efficient electrolyzer achieving ~20 mA cm −2 at a voltage of 1.5 V with good stability was demonstrated. The high activity of NiO/Ni-CNT was possibly attributed to the nanoscopic NiO/Ni interfaces in the heterostructure. The highly active NiO/Ni heterostructure-based catalyst with low cost, earth abundance and environmental friendliness is promising for future water-splitting devices. Oxidization of multi-walled carbon nanotubes MWCNTs were oxidized by a modified Hummers method. MWCNTs (1 g) were purified by calcinations at 500 °C and washing with 40 ml of diluted hydrochloric acid (10 wt%) to remove metal residues and amorphous carbon. The purified MWCNTs were repeatedly washed with water and collected. After drying overnight, ~23 ml of concentrated sulphuric acid was mixed with the purified MWCNTs (~0.99 g) in a 250-ml round flask and stirred at room temperature for 12 h. Subsequently, the round flask was heated to 40 °C in an oil bath, followed by the slow addition of ~100 mg NaNO 3 and ~1 g KMnO 4 (about the same as the mass of purified MWCNTs). After stirring at 40 °C for 30 min, 3 ml of water was added, followed by another 3 ml after 5 min. Water (40 ml) was slowly added 5 min later to keep the temperature below 45 °C. After 15 min, 140 ml of water was poured into the solution at room temperature, followed by the addition of 10 ml of 30% H 2 O 2 to stop the reaction after 10 min. Oxidized MWCNTs were collected, washed with diluted HCl solution (5 wt%) twice and then water repeatedly till pH is higher than or equal to 5. The final suspension (in H 2 O) was lyophilized to get solid oxidized MWCNTs. Synthesis of NiO/Ni-CNT hybrid and control groups In a typical synthesis of NiO/Ni-CNT, ~4 mg oxidized MWCNTs were sonicated in 8 ml of anhydrous N , N -dimethylformamide (DMF) for 10 min, followed by the addition of 800 μl of 0.2 M nickel acetate (Ni(OAc) 2 ) aqueous solution. The mixture was vigorously stirred at 90 °C in an oil bath for 4 h. Afterwards, the suspension was centrifuged and washed with H 2 O twice to get rid of DMF. The resuspended solution was lyophilized to get solid Ni(OH) 2 /ox-CNT. The solid Ni(OH) 2 /ox-CNT was then annealed in a tube furnace at 300 °C and constant pressure of 1.5 torr under Ar atmosphere (100 sccm) for 1 h. The furnace was constantly pumped to get rid of the H 2 O and O 2 generated during the reaction and maintain low pressure in the furnace. After that, the furnace was slowly cooled down to room temperature in ~30 min and the NiO/Ni-CNT catalyst was taken out and ready for use. Ni/CNT was synthesized by the same procedure with raised temperature to 500 °C for the annealing process. NiO/CNT was synthesized by the same procedure with no pumping (400 sccm Ar atmosphere, ~1 atm pressure) for the annealing process. Pure nanoparticles were synthesized by typical procedures of NiO/Ni-CNT synthesis without CNT precursors. Synthesis of NiFe LDH nanoparticles In a typical procedure, 160 μl of 0.5 M Ni(OAc) 2 aqueous solution and 32 μl of 0.5 M Fe(NO 3 ) 3 were mixed with 4 ml DMF by stirring. The mixture was heated to and maintained at 120 °C for 16 h in an autoclave. The temperature was then raised to 160 °C for 2 h. After cooling down to room temperature, the sample was collected, centrifuged, washed with water and finally lyophilized to get solid NiFe LDH nanoparticles. Materials characterizations XPS samples were drop dried onto silicon substrate and measured on a PHI VersaProbe Scanning XPS Microprobe. STEM imaging and EELS mapping was performed on a Nion UltraSTEM-100, operated at 60 kV. XANES measurements were carried out at the SGM beamline of the Canadian Light Source. XANES were measured on indium foil in the surface sensitive total electron yield. Before sample measurement, data were first normalized to the incident photon flux I0 measured with a refreshed gold mesh. After measurement, data were further normalized to the edge jump between pre-edge platform and post-edge platform. Sample preparation for electrochemical measurement To prepare the NiO/Ni-CNT on RDE electrode, 1 mg NiO/Ni-CNT hybrid was mixed with 190 μl water, 50 μl ethanol and 10 μl 5 wt% Nafion solution by at least 30 min sonication to form a homogeneous ink. Subsequently, 20 μl suspension was drop dried onto a glassy carbon electrode of 5 mm in diameter (loading of 0.40 mg cm −2 including CNTs and loading of 0.28 mg cm −2 for the active mass). To prepare the NiO/Ni-CNT on Ni foam electrode, Ni(OH) 2 /ox-CNT was collected after 90 °C oil bath process and washed with ethanol once. Ni(OH) 2 /ox-CNT was then redispersed in ~2 ml ethanol. After sonication for 10 min, all suspension was drop dried onto 1 × 1 cm Ni foam (1.6-mm thick, 100 p.p.i., 95% porosity, Marketech) at 90 °C. The electrode was further heated at 120 °C for ~20 min till fully dry. The as-prepared electrode was annealed in a tube furnace at 300 °C and constant pressure of 1.5 torr under Ar atmosphere (100 sccm) for 1 h, same as typical procedure. The electrode with catalyst was ready for use after the annealing. The loading of NiO/Ni-CNT was determined to be ~11 mg cm −2 by the difference of the weight of Ni foam before and after loading and the active mass was determined to be ~8 mg cm −2 excluding the mass of CNT. The NiFe LDH on Ni foam electrode was produced by drop drying 8 mg NiFe LDH (in 2 ml ethanol+3 wt% PTFE) onto 1 cm × 1 cm Ni foam. Electrochemical measurement HER catalytic activity measurement was performed in a standard three-electrode system controlled by a CHI 760D electrochemistry workstation. Catalyst powders cast on RDE or Ni foam was used as working electrode, graphite rod as counter electrode and saturated calomel electrode as reference electrode. The reference was calibrated against and converted to reversible hydrogen electrode (RHE). RDE electrode was constantly rotating at 1,600 r.p.m. to get rid of the bubbles during the measurement. Water electrolysis measurement was carried out in a standard two-electrode system by using NiO/Ni-CNT on Ni foam as cathode and NiFe LDH on Ni foam as anode. Linear sweep voltammetry was carried out at 1 mV s −1 for the polarization curves. Chronopotentiometry was measured under a constant current density of 20 mA cm −2 . All polarization curves were iR corrected. How to cite this article: Gong, M. et al. Nanoscale nickel oxide/nickel heterostructures for active hydrogen evolution electrocatalysis. Nat. Commun. 5:4695 doi: 10.1038/ncomms5695 (2014).